Rotated waveplates in integrated waveguide optics Controlling and manipulating the polarization state of a light beam is crucial in applications ranging from optical sensing to optical communications, both in the classical and quantum regime, and ultimately whenever interference phenomena are to be exploited. In addition, many of these applications present severe requirements of phase stability and greatly benefit from a monolithic integrated-optics approach. However, integrated devices that allow arbitrary transformations of the polarization state are very difficult to produce with conventional lithographic technologies. Here we demonstrate waveguide-based optical waveplates, with arbitrarily rotated birefringence axis, fabricated by femtosecond laser pulses. To validate our approach, we exploit this component to realize a compact device for the quantum state tomography of two polarization-entangled photons. This work opens perspectives for integrated manipulation of polarization-encoded information with relevant applications ranging from integrated polarimetric sensing to quantum key distribution. Polarization of light is widely adopted as information carrier in a wealth of photonic applications; to cite just a few examples one can mention polarimetric sensing [1] and imaging [2] , or advanced techniques for increasing bandwidth in optical communications such as polarization division multiplexing [3] . The polarization degree of freedom is also broadly exploited in the quantum information field: two orthogonal polarization states of single photons are often adopted as two levels to encode qubits (the so-called polarization encoding), with applications including quantum computing [4] , quantum simulation [5] and quantum communication [6] , [7] . A waveguide optics architecture may offer its striking advantages in terms of intrinsic interferometric stability and compactness to all these applications. However, controlling and manipulating the polarization state of light propagating in an optical waveguide is, in general, not trivial. In particular, producing integrated waveplates with arbitrary optical axis direction is a challenging task with conventional waveguide fabrication technologies, because these components require altering the waveguide symmetry in the three dimensions [8] , [9] , [10] , which is not easy with lithographic techniques. Femtosecond laser writing [11] is an alternative waveguide fabrication technology, which, in the recent years, has been evolving from the proof-of-principle stage [12] to a valid approach for fabricating complex circuits [13] , [14] . This technique exploits non-linear absorption of focused ultrashort pulses to create localized regions with increased refractive index in the volume of dielectric substrates. Translation of the sample at constant speed under the laser beam allows to literally draw three-dimensional waveguiding paths with the desired design. This unique three-dimensional capability represents a remarkable advantage of femtosecond laser direct writing over lithographic techniques, together with the possibility of rapid prototyping of new devices with low production costs. The low birefringence of the fabricated waveguides, when certain irradiation parameters are used, has recently led to the development of femtosecond-laser-written optical circuits able to operate and manipulate different polarization states, in particular able to support polarization-entangled photons for quantum optics applications [15] . Polarization-dependent [16] , [17] or -independent [5] directional couplers have been also reported, bringing to the realization of an integrated polarization-based quantum logic gate [17] , as well as complex interferometric structures for quantum simulation [18] . In fact, integrated waveplates with arbitrary axis direction, which effectively allow one to rotate arbitrarily the polarization state of a propagating photon, have never been reported by femtosecond laser writing. Fernandes et al . [19] , [20] showed in recent works that the birefringence of femtosecond-laser-written waveguides can be finely tuned in fused silica substrate and, in particular, they demonstrated highly controlled integrated linear retarders. However, in those works the optical axis of the birefringent waveguides was fixed along the vertical or horizontal direction. In this work, we develop a method to fabricate integrated waveguide waveplates with tilted axis, by femtosecond laser writing. As we will show, our method requires an extremely simple experimental apparatus. We prove the potential of this technology by realizing and successfully testing a compact device for quantum state tomography (QST) [21] of two polarization-entangled photons. Method for writing rotated waveguides Femtosecond-laser-written waveguides are slightly birefringent (typical values range in b =10 −5 ÷10 −4 ), that is, they support guided modes with different propagation constants for two orthogonal polarization states. The microscopic causes of this birefringence may be diverse depending on the substrate material and the irradiation conditions: ellipticity of the waveguide cross-section [22] , mechanical stress in the modified region [23] or laser-induced intrinsic birefringence aligned according to the writing beam polarization [24] . We experimentally verified that in the boro-aluminosilicate glass, which we use to produce integrated quantum photonic circuts [15] , the polarization direction of the writing laser beam does not affect the waveguide birefringence. Thus, in this glass, we expect only the first two mechanisms to be effective. In this view the waveguide writing process presents an evident symmetry constraint: considering a Gaussian writing beam, a single-pulse modification will have a rotational symmetry with respect to the writing beam direction. Hence, independently of the specific microscopic causes of the birefringence, the optical axis will be parallel to this direction. In the vast majority of the waveguide writing experiments reported in the literature, the laser beam direction is orthogonal to the substrate surface and the writing is performed by scanning the beam transversely to its direction ( Fig. 1a ). The waveguide optical axis is therefore typically orthogonal to the sample surface. Accordingly, the easiest way to tilt the waveguide optical axis would be to rotate the writing beam of an angle θ with a rotation axis parallel to the waveguide direction. In this way the waveguide cross-section, together with its optical axis, would rotate of the same angle θ . However, a macroscopic rotation of the glass with respect to the writing laser beam, or vice versa, would not be a convenient solution. In fact, to avoid large translations of the writing beam inside the glass sample at every rotation θ , a hard-to-obtain resolution in setting the position of the rotation axis would be required. In addition, light refraction at the tilted glass interface would further complicate the fine positioning of the writing focal spot. Finally, the angle-dependent aberrations and Fresnel reflections of the writing beam across the tilted glass interface would make it necessary to re-optimize the laser irradiation parameters for each tilt angle. 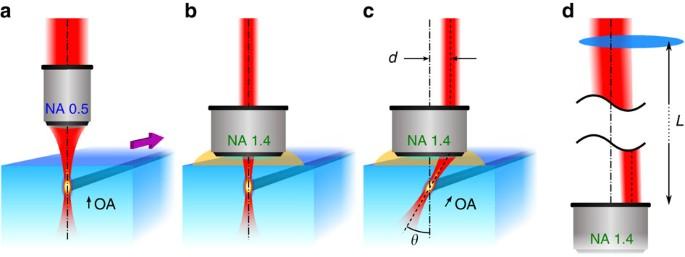Figure 1: Femtosecond laser writing of tilted integrated waveplates. Conceptual scheme of the method enabling the direct writing of optical waveguides acting as integrated waveplates with tilted axis. (a) Traditional writing scheme adopting a focusing objective with moderate NA; the symmetry of the writing layout creates birefringent waveguides with the optical axis (OA) aligned as the writing beam direction; actual waveguide writing is performed by a transverse translation of the glass sample (indicated by the purple arrow). (b) Equivalent waveguides can be created by underfilling a high-NA oil-immersion objective. (c) Offsetting the writing beam before the objective results in waveguide writing with an inclined laser beam; the resulting waveguide has an optical axis tilted by an angleθthat depends on the amount of offsetdof the writing beam with respect to the objective axis. (d) Reduced beam size and offset at the objective aperture is achieved by a small transverse shift of a long focal lens placed at a distanceLfrom the focusing objective (see Methods for details). Figure 1: Femtosecond laser writing of tilted integrated waveplates. Conceptual scheme of the method enabling the direct writing of optical waveguides acting as integrated waveplates with tilted axis. ( a ) Traditional writing scheme adopting a focusing objective with moderate NA; the symmetry of the writing layout creates birefringent waveguides with the optical axis (OA) aligned as the writing beam direction; actual waveguide writing is performed by a transverse translation of the glass sample (indicated by the purple arrow). ( b ) Equivalent waveguides can be created by underfilling a high-NA oil-immersion objective. ( c ) Offsetting the writing beam before the objective results in waveguide writing with an inclined laser beam; the resulting waveguide has an optical axis tilted by an angle θ that depends on the amount of offset d of the writing beam with respect to the objective axis. ( d ) Reduced beam size and offset at the objective aperture is achieved by a small transverse shift of a long focal lens placed at a distance L from the focusing objective (see Methods for details). Full size image We therefore developed a technique to obtain a birefringent waveguide with tilted optical axis without the drawbacks of a macroscopic rotation of the sample with respect to the writing laser beam. Typical waveguide writing is performed with moderate numerical aperture (NA) microscope objectives (for example, NA=0.5, Fig. 1a ) to achieve the required waveguide size in a single scan. Our new method to tilt the waveguide optical axis is based on a high-NA oil-immersion objective (typical NA=1.4, Fig. 1b ) and a writing laser beam with a diameter smaller than the objective aperture. The reduced dimension of the laser beam with respect to the objective aperture is responsible for a reduced effective NA of the oil-immersion objective. An optimization of the beam size can yield an effective NA producing the same waveguides one would obtain with the dry, moderate NA objective ( Fig. 1a,b ). If the laser beam impinges on the centre of the objective, the beam propagates (orthogonally to the substrate surface) without changing its direction. If the laser beam impinges on the objective aperture in an off-centre way, the focus position is not altered, but the beam propagates in the substrate at an angle θ that depends on the offset distance on the objective (see Fig. 1c ). The fabricated waveguide will then have a tilted cross-section, resulting in a rotated optical axis. One can observe that being the focus position independent from the beam offset at the aperture (which is true for any commercial, aberration-compensated microscope objective), the position of the fabricated waveguide is always the same, for any angle θ . In addition, as the objective remains always orthogonal to the substrate surface, the aberrations are well compensated, while the presence of the immersion oil quenches the Fresnel reflections at the glass interface. This means that the pulse energy delivered at the focal spot is always the same for any θ and no adjustment is required. As well, the use of immersion oil eliminates the aberrations given by the air–glass interface, enabling the fabrication of waveguides with negligible dependence of their properties on the depth (see Supplementary Fig. 1 ). Tilting of the writing beam inside the glass requires a transverse offset of the beam before the focusing objective. This could be effectively done with a pair of motorized mirrors. In our set-up, however, we implemented a very simple variant, based on a single, long-focal lens mounted on a linear translator ( Fig. 1d ). The lens, mounted before the focusing objective, has the twofold effect of reducing the beam diameter to achieve the reduced effective NA and, at the same time, to shift the incidence point on the objective aperture by a small transverse translation of the lens. In fact, this is not a pure translation of the beam impinging on the objective, as it also adds an angular deviation. The latter deviation is however very small given the long focal length and the limited objective aperture. A careful analysis showed that the angular deflection introduced by the lens results in a shift in the writing focal point in the order of a few micrometres. This shift is very reproducible and can be easily compensated during the waveguide writing process. Details on the experimental set-up can be found in the Methods section, Supplementary Fig. 2 and Supplementary Note 1 . Characterization of rotated waveguides as integrated waveplates As a first experiment we fabricated several waveguides with different tilt angles produced by different shifts of the long-focal lens before the focusing objective. For each fabricated waveguide we measured the tilt angle of its cross-section, by acquiring images of the waveguide end-facet with an optical microscope (see Fig. 2a and Supplementary Fig. 3 ). To fully characterize the waveguide birefringence we measured the Stokes vector of the output polarization state when launching several different input polarization states; we then retrieved the value of birefringence and the optical axis tilt angle that best fitted the experimental data for each waveguide. As shown in Table 1 , we found a very good agreement between the tilt angle of the cross section, retrieved by the microscope images and the tilt angle of the optical axis determined by the polarization analysis. This confirms our idea that rotating the waveguide cross-section implies a rotation of the optical axis of the same angle. It should be observed that the maximum tilting angle achievable with this technique is limited by the NA of the microscope objective. In our set-up with NA=1.4, we achieved rotations of the optical axis up to 27° with respect to the vertical axis (not limiting arbitrary operations on the polarization state, as shown in Supplementary Note 2 ). In addition, we observe that the birefringence value b remains essentially the same at all the different angles with an average . Finally, we measured the near-field profile of the guided mode at 800 nm wavelength for each waveguide ( Fig. 2b ), noting no relevant differences in the mode size and shape. This confirms that our technique is able to rotate the optical axis with negligible effect on all the other waveguide features. This very important property implies low insertion losses in practical devices, where waveguides with different optical axis direction will be written consecutively. 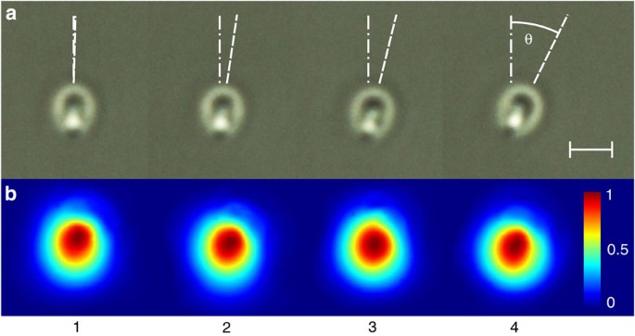Figure 2: Experimental characterization of tilted waveguides. (a) End-view microscope images of waveguides (labelled 1–4) showing a progressive rotation of the cross-section as the offsetdof the writing beam is increased. Scale bar, 5 μm. (b) Near-field profiles of the waveguide modes at different rotation angles. Quantitative measures are reported inTable 1. Figure 2: Experimental characterization of tilted waveguides. ( a ) End-view microscope images of waveguides (labelled 1–4) showing a progressive rotation of the cross-section as the offset d of the writing beam is increased. Scale bar, 5 μm. ( b ) Near-field profiles of the waveguide modes at different rotation angles. Quantitative measures are reported in Table 1 . Full size image Table 1 Relevant parameters of the waveguides with a tilted optical axis. Full size table To cascade waveguide segments with different orientations of the optical axis we write the different segments in successive scans. This is made possible by a mechanical shutter synchronized with the motion of the translation stages; the shutter enables the irradiation only in the regions where waveguide segments with a given optical axis tilt have to be fabricated. Next, the long focal lens is translated to a new position and the segments with a different optical axis tilt are produced. 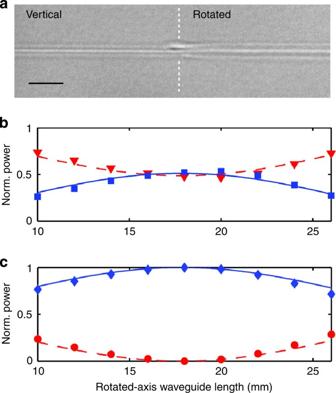Figure 3: Characterization of integrated optical waveplates. (a) Top-view microscope image of a junction between two waveguide sections having different tilt angles. Scale bar, 10 μm. Several waveplates with a designed optical axis tilt ofθ=22.5° with different lengths have been characterized; for horizontally polarized input light, the measured normalized power transferred into (b) the horizontal (red triangles)/vertical (blue squares) polarization states and (c) diagonal (blue diamonds)/antidiagonal (red circles) polarization states is reported. Error bars are omitted, as they are smaller than the symbols. Theoretical curves best fitting the experimental points are plotted and correspond toθ=21.5°, consistent with the accuracy of our fabrication method in setting the tilt angle, estimated asσθ=1.5°. Figure 3 shows a microscope top-view image of the junction between two waveguide segments with different optical axis direction; a perfect alignment can be appreciated, while the slight discontinuity causes only 0.3 dB additional losses. To test our capability to fabricate effective integrated waveplates we realized waveguides comprising two segments: the first with vertical optical axis and the second with optical axis tilted by 22.5°. Keeping constant the overall length of the waveguide, we varied the length of the two segments. We characterized the devices by injecting horizontally and vertically polarized laser light into the segment with a vertical optical axis and by measuring the projections on the vertical (V), horizontal (H), diagonal (D) and antidiagonal (A) polarization states of the output (see, for example, Fig. 3b,c for H polarized input state projected onto the H/V and D/A bases, respectively). The first waveguide segment has actually no influence on the vertical or horizontal input polarization states, while the second one introduces a polarization rotation. The induced polarization rotations fit very well with the theoretical behaviour calculated for the different lengths of the segment with rotated axis. At a suitable length of ~18 mm of the second segment a clear half-waveplate operation is observed: >99% of the incoming H polarized light is converted into D polarization state. Coherently, no light is found in the A state, while an even splitting of light is found in the H/V basis. Figure 3: Characterization of integrated optical waveplates. ( a ) Top-view microscope image of a junction between two waveguide sections having different tilt angles. Scale bar, 10 μm. Several waveplates with a designed optical axis tilt of θ =22.5° with different lengths have been characterized; for horizontally polarized input light, the measured normalized power transferred into ( b ) the horizontal (red triangles)/vertical (blue squares) polarization states and ( c ) diagonal (blue diamonds)/antidiagonal (red circles) polarization states is reported. Error bars are omitted, as they are smaller than the symbols. Theoretical curves best fitting the experimental points are plotted and correspond to θ =21.5°, consistent with the accuracy of our fabrication method in setting the tilt angle, estimated as σ θ =1.5°. Full size image Integrated device for QST As a probing benchmark of our technology, we fabricated the complex device represented in Fig. 4a , which is an integrated optical analyser of two-photon polarization states. The device is composed of two twin parts, one per each photon (A and B). Each part comprises a network of polarization-independent couplers (we employed the three-dimensional architecture devised in ref. 5 ) that equally split the input light into three arms. The α -arm consists in a waveguide with vertical birefringence axis. The β -arm ends with a waveguide segment operating as a half-waveplate, tilted by 22.5° (the remaining segment with tilt 0° does not have any effect on the polarization measurement, as its optical axis is aligned to the polarizing beam splitter (PBS) placed at the output, see Fig. 4b ). The γ -arm ends with two consecutive waveguide segments, acting as a vertically oriented quarter waveplate and a half-waveplate tilted by 22.5°. The polarization rotations induced by the input fibres and by the first part of the integrated device (up to the dashed line in Fig. 4a ) are compensated by fibre polarization controllers in each input mode ( Fig. 4b ). By cascading to this device a single (bulk) polarization beam splitter it is possible to achieve a parallel analysis of the polarization state of the input light in the three bases (vertical and horizontal, diagonal and antidiagonal, right- and left-handed circular polarization). Hence, a complete tomography of one- and two-photon polarization states can be accomplished. 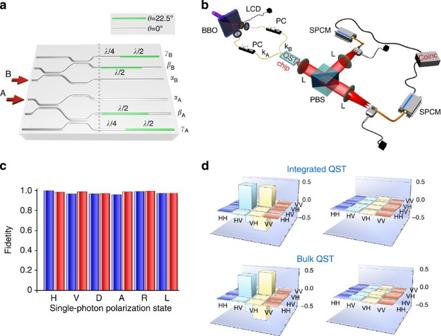Figure 4: QST in an integrated chip. (a) Scheme of the integrated device (QST chip) for quantum tomography of a two-photon state: it is composed of two specular circuits, one for photon A and one for photon B; these circuits, by means of integrated waveplates of suitable length and tilt, prepare the two-photon state to have it projected on the horizontal (H)/vertical (V), diagonal (D)/antidiagonal (A) and circular left (L)/circular right (R) bases by a single PBS placed afterwards (see set-up inb). (b) Scheme of the experimental set-up for the tomography of entangled states (for details see Methods). (c) Fidelities for quantum tomography of different single-photon polarization states; blue and red bars represent the results obtained by input of the same polarization state in A and B modes, respectively. Error bars are omitted as they were too small compared with the axis scale. (d) Real (left) and imaginary (right) part of the reconstructed density matrix for a polarization-entangled Bell state (Ψ−); comparison is shown between the measurement made with the integrated chip and that performed by a standard QST set-up with bulk optical elements. Figure 4c,d shows the results of our measurements with single- and two-photon states (technical details in the Methods and Supplementary Note 3 ). In particular, Fig. 4c reports the fidelities of the tomographic measurements on single-photon states, with an average value of 0.976±0.03 (fidelity for each single-photon state is reported in Supplementary Table 1 ). Figure 4d shows the reconstructed density matrix of a polarization-entangled Bell state, which yields a 0.971±0.006 fidelity to the same measurement performed with a standard bulk-optics QST equipment. Figure 4: QST in an integrated chip. ( a ) Scheme of the integrated device (QST chip) for quantum tomography of a two-photon state: it is composed of two specular circuits, one for photon A and one for photon B; these circuits, by means of integrated waveplates of suitable length and tilt, prepare the two-photon state to have it projected on the horizontal (H)/vertical (V), diagonal (D)/antidiagonal (A) and circular left (L)/circular right (R) bases by a single PBS placed afterwards (see set-up in b ). ( b ) Scheme of the experimental set-up for the tomography of entangled states (for details see Methods). ( c ) Fidelities for quantum tomography of different single-photon polarization states; blue and red bars represent the results obtained by input of the same polarization state in A and B modes, respectively. Error bars are omitted as they were too small compared with the axis scale. ( d ) Real (left) and imaginary (right) part of the reconstructed density matrix for a polarization-entangled Bell state (Ψ − ); comparison is shown between the measurement made with the integrated chip and that performed by a standard QST set-up with bulk optical elements. Full size image In summary, we have developed a technique to fabricate waveguide segments acting as integrated waveplates, with precise control of the tilt angle. Our approach is much simpler and cost-effective than other lithography-based techniques to realize integrated polarization converters. We demonstrate the capability of our devices to perform arbitrary transformations on the polarization state of light propagating in an integrated waveguide circuit, with both classical and quantum states of light. In particular, an integrated device for the analysis of the polarization state of two entangled photons is provided. The scope of the present device was to demonstrate the quality of our integrated waveplates in a relevant and demanding application. For this reason the PBS was kept as a bulk element to clearly isolate the role of the integrated waveplates with respect to a standard all-bulk set-up. Nevertheless, the possibility to achieve a fully integrated QST device is very intriguing. As a perspective, a PBS could be integrated following the same scheme already presented in refs. 16 , 17 . The combination of these components should enable the demonstration of a fully integrated QST chip. Future work will aim at reducing the footprint of these devices by locally enhancing the waveguide birefringence (for example, using the approach proposed in ref. 20 ). This work opens the way to the integration of a broader set of experiments and devices that use photon polarization, including on-chip classical polarimetry [25] , on-chip quantum metrology [26] , as well as the integrated manipulation of hyperentangled photon states [27] . Femtosecond laser waveguide writing Our waveguide fabrication set-up is based on a regeneratively amplified Yb:based femtosecond laser system (HIGHQLaser FemtoREGEN), with wavelength λ =1,040 nm, pulse duration of 400 fs and 960 kHz repetition rate. The beam is focused by an NA=1.4 oil-immersion microscope objective, at 170 μm depth below the surface of borosilicate glass substrates (Corning EAGLE 2000). Sample translation at constant speed is provided by Aerotech FiberGLIDE high-precision, air-bearing translation stages. To deflect the laser beam and translate its incidence point on the objective aperture, a spheric lens with focal length f =50 cm was used, located at a distance L =44 cm from the objective aperture. This allowed us to reduce the laser spot size to a 1/ e 2 diameter 2 w =1.6 mm, which is ~2.8 times smaller than the objective aperture D =4.5 mm. The effective NA approximately scales by the same factor with respect to the full value NA=1.4, reaching an NA eff ~0.5, which is comparable to values commonly employed for femtosecond laser waveguide writing. With the configuration detailed above, we were able to fabricate waveguides with a maximum tilt angle of the birefringence axis of 27°. By further reducing the spot size on the objective aperture we achieved a maximum angle of 45° (see Supplementary Fig. 4 and Supplementary Note 1 ); however, the latter condition required working at the edge of the objective aperture, thus being less reliable. A mechanical shutter (Thorlabs SH05) is used to juxtapose different waveguide segments written with different optical axis directions. Optimum single-mode waveguides at 800 nm were fabricated with a pulse energy of 210 nJ and translation speed of 20 mm s −1 . Propagation losses at 800 nm wavelength have been measured as 0.2 dB cm −1 . The whole chip for tomography yields additional insertion losses (including coupling losses, propagation and bending losses) of 4.4 dB for a 5-cm-long device. Coupling losses due to mismatch between fibre and waveguide modes have been estimated as 0.7 dB, from a numerical overlap integral of the mode profiles. Measurements with quantum light Let us refer to Fig. 4b . To perform measurements with quantum light, a β -barium borate crystal cut for type II phase matching and pumped by a continuous-wave diode laser ( λ =405 nm) generates polarization-entangled photon pairs in the state at λ =810 nm via spontaneous parametric down conversion [28] . Photon pairs are then delivered to the integrated circuit (QST chip) through single-mode fibres. The output modes of the chip are collected by an aspheric lens (L) and delivered to a bulk PBS, which transmits horizontal and reflects vertical polarized light. Both the transmitted and the reflected modes are collected by multimode fibres mounted on motorized stages. Photons are then detected by single-photon-counting modules and coincidences between photon pairs are finally recorded. Birefringence compensation The waveguides constituting the first part of the fabricated device for QST are birefringent, and some birefringence is also present unavoidably in the optical fibres used to inject photons in the chip. To compensate for the polarization rotations induced by the propagation in these sections of the circuit (fibres and waveguides) we adopted the following strategy. First, we compensated horizontal and vertical polarization by means of standard polarization controllers acting on the input fibres, by injecting horizontally polarized light and measuring the state emerging from the α outputs (see Fig. 4a ). Second, we adjusted the phase between horizontal and vertical polarizations with a liquid-crystal controllable waveplate, by injecting into the chip diagonal (circular) polarized light, and measuring the state emerging from the β ( γ ) outputs. How to cite this article: Corrielli, G. et al . Rotated waveplates in integrated waveguide optics. Nat. Commun. 5:4249 doi: 10.1038/ncomms5249 (2014).